Inferring tumour purity and stromal and immune cell admixture from expression data Infiltrating stromal and immune cells form the major fraction of normal cells in tumour tissue and not only perturb the tumour signal in molecular studies but also have an important role in cancer biology. Here we describe ‘Estimation of STromal and Immune cells in MAlignant Tumours using Expression data’ (ESTIMATE)—a method that uses gene expression signatures to infer the fraction of stromal and immune cells in tumour samples. ESTIMATE scores correlate with DNA copy number-based tumour purity across samples from 11 different tumour types, profiled on Agilent, Affymetrix platforms or based on RNA sequencing and available through The Cancer Genome Atlas. The prediction accuracy is further corroborated using 3,809 transcriptional profiles available elsewhere in the public domain. The ESTIMATE method allows consideration of tumour-associated normal cells in genomic and transcriptomic studies. An R-library is available on https://sourceforge.net/projects/estimateproject/ . Malignant solid tumour tissues consist of not only tumour cells but also tumour-associated normal epithelial and stromal cells, immune cells and vascular cells. Stromal cells are thought to have important roles in tumour growth, disease progression [1] , [2] and drug resistance [3] . Infiltrating immune cells act in a context-dependent manner, and whereas antitumor effects of infiltrating T-lymphocytes have been observed in ovarian cancer [4] , [5] , [6] , associations with tumour growth, invasion and metastasis were described in colorectal cancer [7] , [8] . The comprehensive understanding of tumour-associated normal cells in tumour tissues may provide important insights into tumour biology and aid in the development of robust prognostic and predictive models. Gene expression profiling of cancer has resulted in the identification of molecular subtypes and the development of models for prediction prognosis and has enriched our knowledge of the molecular pathways of tumorigenesis [9] , [10] , [11] , [12] , [13] . Increasing evidence suggests that the infiltration of tumour-associated normal cells influences the analysis of clinical tumour samples by genomic approaches, such as gene expression profiles or copy number data, and biological interpretation of the results requires considerable attention to sample heterogeneity [14] , [15] , [16] . Several methods have been proposed to estimate the fraction of tumour cells in clinical tumour samples by using DNA copy number array data [14] , [15] or by using next-generation sequencing data [17] . DNA copy number-based estimation of tumour purity is rapidly gaining traction in predicting the purity of tumour samples; however, such methods are limited to samples with available copy number profiles. Previous studies have attempted to deconvolve gene expression data into gene expression profiles from their constituent cellular fractions, whereas others have focused on deconvolution of microarray data obtained from normal tissue into cell-type-specific profiles, by calculating enrichment scores [18] , [19] , [20] , [21] , [22] . These methods take advantage of the differences in transcriptome properties of distinct cell types. Here we present a new algorithm that takes advantage of the unique properties of the transcriptional profiles of cancer samples to infer tumour cellularity as well as the different infiltrating normal cells, called ESTIMATE (Estimation of STromal and Immune cells in MAlignant Tumour tissues using Expression data). We focus on stromal and immune cells that form the major non-tumour constituents of tumour samples and identify specific signatures related to the infiltration of stromal and immune cells in tumour tissues [1] . By performing single-sample gene set-enrichment analysis (ssGSEA) [13] , [23] , we calculate stromal and immune scores to predict the level of infiltrating stromal and immune cells and these form the basis for the ESTIMATE score to infer tumour purity in tumour tissue. Finally, we describe the biological characteristics of stromal and immune scores in The Cancer Genome Atlas (TCGA) data sets [24] , [25] , [26] , [27] , [28] , [29] . Estimation of infiltrating cells and tumour purity An overview of ESTIMATE algorithm is shown in Fig. 1 . We devised two gene signatures: (1) a ‘stromal signature’ that was designed to capture the presence of stroma in tumour tissue, and (2) an ‘immune signature’ that aimed to represent the infiltration of immune cells in tumour tissue ( Supplementary Data 1 ). To generate these signatures, we performed the following steps ( Fig. 1 ). Genes associated with the quantity of infiltrating immune cells in tumour tissue were identified using leukocyte methylation scores, which were previously shown to correlate with the presence of leukocytes in ovarian carcinomas [15] . Gene expression profiles of normal hematopoietic samples were compared with those of other normal cell types. The overlap between the two gene sets constituted the immune signature. Stromal-related genes were selected among non-hematopoiesis genes by comparison of the tumour cell fraction and matched stromal cell fraction after laser-capture microdissection in breast, colorectal and ovarian cancer data sets [30] , [31] , [32] . Genes with high variability in cancer cell lines and genes highly expressed in glioma stem-like cells were filtered to make up the stromal signature. We used single-sample ssGSEA [13] , [23] of these two signatures to generate scores that reflect the presence of each cell type in tumour samples and combined represent a measurement of tumour purity. 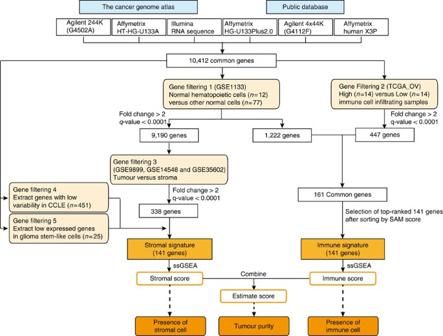Figure 1: An overview of the ESTIMATE algorithm. The ESTIMATE algorithm uses gene expression data to output the estimated levels of infiltrating stromal and immune cells and estimated tumour purity. Infiltrating stromal- and immune cell-related genes were identified by five gene filterings. Figure 1: An overview of the ESTIMATE algorithm. The ESTIMATE algorithm uses gene expression data to output the estimated levels of infiltrating stromal and immune cells and estimated tumour purity. Infiltrating stromal- and immune cell-related genes were identified by five gene filterings. Full size image In order to evaluate the reliability of the stromal and the immune signatures, we obtained three ovarian carcinoma tumour samples and performed microbead-based cell sorting to separate tumour and non-tumour cell fractions. The epithelial, tumour cell-containing, cell fraction was enriched using an EpCAM antibody. Transcriptional profiles were obtained from the bulk tumour samples as well as the EpCAM-positive and EpCAM-negative cell fractions. Although tumour cells may not necessarily express EpCAM and some normal epithelial cells may express EpCAM [33] , a significant reduction in stromal signature scores (paired t- test, P =0.0042) and a declining trend in immune signature scores (paired t- test, P =0.072) were observed in all three EpCAM-positive cell fractions compared with the EpCAM-negative cell fractions, suggesting that these signatures are associated with the amount of non-epithelial cells in tumour samples ( Fig. 2a ). 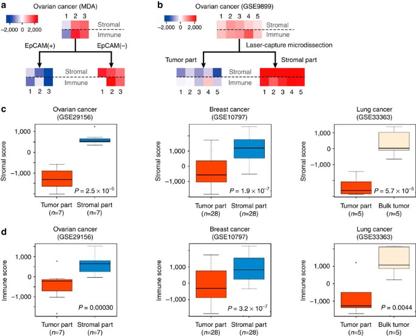Figure 2: Stromal and immune scores for tumour cell and stromal fractions of tumour samples. Stromal and immune scores were generated using expression data sets obtained from tumour cell or stromal cell-enriched samples. (a,b) Heatmaps display stromal (upper row) and immune score (lower row) per sample (each column) using ovarian cancer samples after (a) microbead-based cell sorting and (b) laser-capture microdissection (red=high, blue=low score). (c,d) Box and whisker plots display reduced (c) stromal and (d) immune scores for the tumour cell-enriched samples (tumour part) after laser-capture microdissection compared with matched stromal cell-enriched (ovary, breast) or bulk tumour samples (lung). Box represents the median (thick line) and the quartiles (line). Whisker expresses 1.5 interquartile range (IQR) of the lower or the upper quartile. Figure 2: Stromal and immune scores for tumour cell and stromal fractions of tumour samples. Stromal and immune scores were generated using expression data sets obtained from tumour cell or stromal cell-enriched samples. ( a , b ) Heatmaps display stromal (upper row) and immune score (lower row) per sample (each column) using ovarian cancer samples after ( a ) microbead-based cell sorting and ( b ) laser-capture microdissection (red=high, blue=low score). ( c , d ) Box and whisker plots display reduced ( c ) stromal and ( d ) immune scores for the tumour cell-enriched samples (tumour part) after laser-capture microdissection compared with matched stromal cell-enriched (ovary, breast) or bulk tumour samples (lung). Box represents the median (thick line) and the quartiles (line). Whisker expresses 1.5 interquartile range (IQR) of the lower or the upper quartile. Full size image In the three data sets used in the process of gene selection, there was a significant reduction in the stromal and immune scores in the tumour cell fraction ( Fig. 2b ; Supplementary Fig. S1 ). Similarly, the microdissected stroma-enriched fraction in the three independent public data sets, which were not used in construction of the gene signature was significantly decreased (ovarian cancer (GSE29156), P =2.5 × 10 −5 ; breast cancer (GSE10797), P =1.9 × 10 −7 ; lung cancer (GSE33363), P =5.7 × 10 −7 by paired t- test; Fig. 2c ). Although immune scores in the tumour cell-enriched fraction were lower than those in bulk tumour- or stroma-enriched fraction (ovarian cancer, P =0.0030; breast cancer P =3.2 × 10 −7 ; lung cancer P =0.0044 by paired t -test; Fig. 2d ), one tumour-enriched sample retained a high immune score ( Fig. 2b ), suggesting that immune cells were retained in the microdissected tumour cell-enriched fraction. This observation may reflect the challenges in microdissecting tumour and immune cells that intermix in many tumours. It could also be related to differences between infiltrating immune cells and immune cells surrounding the tumour [4] , [5] , [6] . To evaluate the association of the stromal and immune scores with tumour purity, we compared ESTIMATE scores with predictions of tumour purity based on the ABSOLUTE method [15] . ABSOLUTE establishes the fraction of tumour cells in a tumour sample based on somatic DNA copy number alterations and has been shown to provide highly accurate prediction of tumour purity. Immune and stromal signature scores of TCGA Agilent array-based expression profiles of ovarian cancer ( n =417; 28 samples used to define the immune signature were not included in this analysis) showed a significant correlation of both stromal and immune scores with ABSOLUTE tumour purity predictions (Pearson’s correlation coefficient or r , −0.65 and −0.60; distance r, 0.65 and 0.58) ( Fig. 3a,b ). Importantly, ESTIMATE scores showed an increased correlation with tumour purity compared with stromal-only and immune-only scores (Pearson’s r , −0.69; distance r , 0.69) ( Fig. 3c ). There was a positive correlation between stromal and immune scores (Pearson’s r , 0.62; distance r, 0.58), and samples with low tumour purity showed high stromal and immune scores ( Fig. 3d ). Specific samples were associated with high stromal but not high immune scores, and vice versa , suggesting variable infiltrating patterns ( Supplementary Data 2 ). 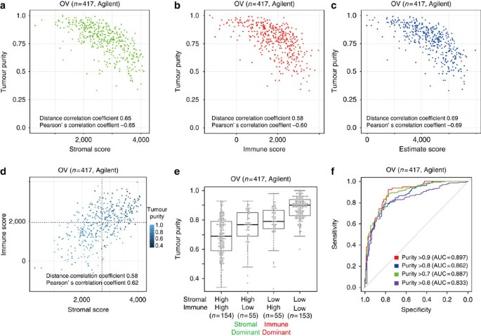Figure 3: The association between tumour purity variables in TCGA’s ovarian cancer data set. (a–d) Scatterplots between tumour purity and (a) stromal, (b) immune, (c) ESTIMATE scores and between (d) stromal and immune scores in the TCGA ovarian cancer data set. TCGA ovarian cancer samples used in the gene selection (n=28) were not included in the figure. Dash lines denote each median value for stromal and immune scores. (e) The association between tumour purity and stromal- or immune-dominant pattern. Four subgroups were divided based on the median of stromal and immune scores. (f) The ROC curves for four cutoff values in TCGA ovarian cancer data set.N=417. Figure 3: The association between tumour purity variables in TCGA’s ovarian cancer data set. ( a – d ) Scatterplots between tumour purity and ( a ) stromal, ( b ) immune, ( c ) ESTIMATE scores and between ( d ) stromal and immune scores in the TCGA ovarian cancer data set. TCGA ovarian cancer samples used in the gene selection ( n =28) were not included in the figure. Dash lines denote each median value for stromal and immune scores. ( e ) The association between tumour purity and stromal- or immune-dominant pattern. Four subgroups were divided based on the median of stromal and immune scores. ( f ) The ROC curves for four cutoff values in TCGA ovarian cancer data set. N =417. Full size image To illustrate the broad utility of the ESTIMATE algorithm, we applied this model to 10 TCGA tumour types for which both DNA copy number and gene expression data sets were available, profiled on four different platforms ( Table 1 ) [24] , [26] , [27] , [28] , [29] . These 10 tumour types were among the first cancers to be characterized by TCGA and were included in TCGA’s Pan-Cancer effort. To confirm the accuracy of the ESTIMATE algorithm, receiver operating characteristic (ROC) curve analysis [34] using ABSOLUTE-based tumour purity was performed. Tumour samples were divided into high- and low-purity groups based on several cutoff values of ABSOLUTE-based tumour purity (0.9, 0.8, 0.7 and 0.6), and the area under the ROC curve (AUC) for each cutoff was measured. For example, a cutoff of 0.7 for tumour purity resulted in Agilent-based ESTIMATE score AUC of 0.89 in the TCGA ovarian cancer data set used as the training set ( Fig. 3f ). Next, we applied the ROC analysis to other data sets by using the same procedure. Similar AUC values were observed across different expression platforms as well as different tumour types ( Fig. 4a ; Supplementary Figs S2–S6 ). Table 1 A list of The Cancer Genome Atlas data sets. 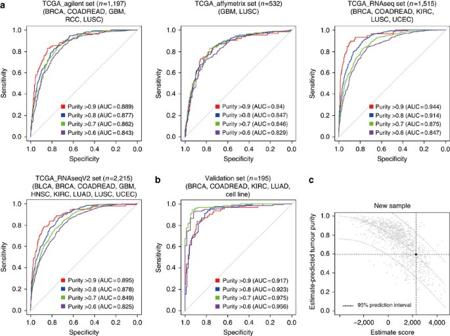Figure 4: Evaluation of ESTIMATE algorithm. The accuracy of the ESTIMATE algorithm was evaluated by the AUC when tumour samples were divided into high- and low-purity groups on the basis of DNA copy number-based tumour purity. (a,b) The ROC curves for four cutoff values in (a) the Agilent data set, the Affymetrix data set, and the RNAseq data set, the RNAseqV2 data set, and (b) the validation data set. (c) An example of ESTIMATE for new Affymetrix sample, with an ESTIMATE-predicted tumour purity of 0.58. Black dot and grey dash lines show ESTIMATE tumour purity and 95% prediction interval, respectively. The grey dots represent the background distribution based on 955 samples from the TCGA Affymetrix data set. Full size table Figure 4: Evaluation of ESTIMATE algorithm. The accuracy of the ESTIMATE algorithm was evaluated by the AUC when tumour samples were divided into high- and low-purity groups on the basis of DNA copy number-based tumour purity. ( a , b ) The ROC curves for four cutoff values in ( a ) the Agilent data set, the Affymetrix data set, and the RNAseq data set, the RNAseqV2 data set, and ( b ) the validation data set. ( c ) An example of ESTIMATE for new Affymetrix sample, with an ESTIMATE-predicted tumour purity of 0.58. Black dot and grey dash lines show ESTIMATE tumour purity and 95% prediction interval, respectively. The grey dots represent the background distribution based on 955 samples from the TCGA Affymetrix data set. Full size image Immune cells not only infiltrate the tumour cell region but have also been demonstrated to associate with stromal cells, in a cancer-type-specific manner [4] . The correlation between stromal and immune scores varied across cancer types, ranging from high (GBM, Pearson’s r =0.8) to modest (KIRC, Pearson’s r =0.38; Fig. 3d ; Supplementary Fig. S7 ). This suggests that the stromal and immune signatures do not measure the same phenotype and reflects the variable association between immune cells and tumour stroma across cancers. Pathology-based estimates of the percentage of tumour cells, stromal cells and infiltrating lymphocytes, evaluated from hematoxylin-eosin-stained slides, were less correlated with ESTIMATE, stromal and immune scores ( Fig. 5 ). 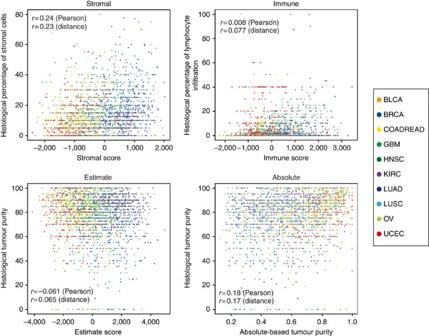Figure 5: Correlation of scores with histological findings. Scatterplots between stromal, immune, ESTIMATE scores and ABSOLUTE-based tumour purity versus the following histological findings: percentage of stromal cells (left upper corner), percentage of infiltrating lymphocytes (right upper corner), and percentage of tumour cells (bottoms panels). Twenty-eight TCGA ovarian cancer samples used in the gene selection were excluded from this analysis. Figure 5: Correlation of scores with histological findings. Scatterplots between stromal, immune, ESTIMATE scores and ABSOLUTE-based tumour purity versus the following histological findings: percentage of stromal cells (left upper corner), percentage of infiltrating lymphocytes (right upper corner), and percentage of tumour cells (bottoms panels). Twenty-eight TCGA ovarian cancer samples used in the gene selection were excluded from this analysis. Full size image Prediction of tumour purity using ESTIMATE In order to facilitate tumour purity prediction using ESTIMATE signatures, we transformed the scoring system to a [0,1] range. First, a regression curve for ESTIMATE score and tumour purity based on ABSOLUTE in the TCGA data set was established. By applying the nonlinear least squares method to the modified TCGA Affymetrix data ( n =995) ( Supplementary Fig. S8a ), ESTIMATE-based tumour purity prediction model was developed. There was a high correlation between ESTIMATE-based and DNA copy number-based tumour purity (Pearson’s r =0.74) ( Supplementary Fig. S8b ). Validating the capacity of ESTIMATE to predict tumour purity was performed using an independent data set ( n =195) composed of seven publicly available data sets including both Affymetrix microarray expression data and matched SNP array copy number data ( Supplementary Table S1 ). Moreover, ESTIMATE-based tumour purities were highly correlated with the ABSOLUTE-based tumour purities in the independent validation set (Pearson’s r =0.87) ( Fig. 4b ; Supplementary Fig. S8c ). When four cutoff values (ABSOLUTE-based tumour purity of 0.9, 0.8, 0.7 and 0.6) were applied, the average and standard deviation of the accuracy per cutoff was 0.87±0.050 ( Supplementary Table S2 ). ESTIMATE provided tumour purity predictions in individual samples with a 95% confidence interval of the validity of the prediction ( Fig. 4c ). To show the specificity of the tumour purity prediction, we used copy number and expression data from 27 cancer cell lines samples (GSE34211). The root-mean-square error of ESTIMATE and ABSOLUTE were 0.006 and 0.051, respectively, indicating consistent absence of immune and stromal signals ( Supplementary Fig. S9 ). Next, we calculated ESTIMATE scores using the expression profiles from 10 normal ovarian epithelium samples (GSE18520). The ESTIMATE-predicted tumour purity was 0.68±0.12 ( Supplementary Table S3 ), suggesting that normal ovarian epithelium may have some stromal or immune cell components. In addition, to clarify whether alteration of gene expression levels related to cell adhesion, migration or wound-healing processes that occur within tumour cells would affect our stromal, immune and ESTIMATE scores, we used public microarray data (GSE17708) from 26 lung adenocarcinoma cell lines treated or untreated by transforming growth factor beta 1. Although our stromal scores slightly increased, the estimated tumour purity was unaffected ( Supplementary Fig. S10 ). We investigated the correlation of the stromal, immune and ESTIMATE scores with methylation-based estimates of the fraction of leukocytes in tumour tissues [15] . A high correlation between our immune score and leukocyte methylation score was observed across all tumour types (Pearson’s r =0.75±0.091) ( Supplementary Fig. S11 ). Interestingly, stromal scores were not strongly correlated with leukocyte methylation score (Pearson’s r =0.51±0.089). These findings showed that our immune scores were specifically associated with the presence of leukocytes across different tumour types. Patterns of stromal and immune cell scores across different tumour types Using both TCGA and non-TCGA data sets from 10 different tumour types ( Supplementary Table S1 ), we examined the distribution of stromal and immune score per tumour type ( Fig. 6 ; Supplementary Fig. S12 , Supplementary Table S4 ). As reported previously, lung adenocarcinomas showed lower purity compared with other tumour types [15] . The relatively high levels of stroma found in clear cell renal cell carcinoma and breast carcinoma may be associated with the high levels of adipocyte content that is characteristic of both tumour types [35] , [36] . In high-grade serous ovarian carcinoma, high stromal or immune scores reflect the presence of mesenchymal or immunoreactive gene expression subtypes that have been reported previously [30] , [37] . Clear cell renal cell carcinomas are considered to be immunogenic tumours, and this characteristic is captured by the relatively high levels of immune signature expression [38] . Immunogenicity is not known as a property of lung squamous cell carcinoma; however, this disease is characterized by a high percentage (>95%) of patients with a history of smoking, which has been linked to lung inflammation [39] , [40] . Lung squamous cell carcinomas showed relatively high immune cell scores and have recently been associated with susceptibility to immunomodulatory therapeutics such as ipilimumab [40] . Further investigation is needed to show that the presence of infiltrating immune cells is a biomarker for immunotherapy response. The similarity in the distribution of stromal and immune scores between lung squamous cell carcinoma and head and neck squamous cell carcinoma suggests that these tumours may harbour a similar genomic profile but also share comparable tumour cellularities [28] . 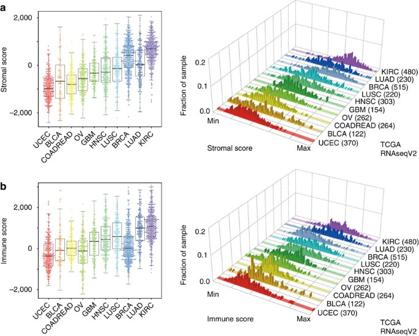Figure 6: Unique distribution of stromal and immune scores. (a,b) Distinct distributions of (a) stromal and (b) immune scores across different tumour types were observed in RNAseqV2Affymetrix platform data sets. The number of parenthesis means sample size per data sets. Figure 6: Unique distribution of stromal and immune scores. ( a , b ) Distinct distributions of ( a ) stromal and ( b ) immune scores across different tumour types were observed in RNAseqV2Affymetrix platform data sets. The number of parenthesis means sample size per data sets. Full size image The impact of tumour purity on somatic mutations To examine the impact of tumour purity on the ability to detect genetic alterations, we assigned samples with ESTIMATE scores in the top 25% to a low-purity subgroup, and samples with the bottom 25% ESTIMATE scores to a high-purity subgroup, per tumour type. We observed a reduced number of mutations per megabase in low-purity head and neck squamous cell carcinomas and clear cell renal cell carcinomas, (unpaired t -test with Benjamini–Hochberg FDR correction, adjusted P =0.055 and 0.055) but not in other tumour types, suggesting that the sequencing coverage used for TCGA samples is sufficient to comprehensively detect somatic sequence variants ( Supplementary Fig. S13 ). Next, we evaluated the mutation spectrum of high- and low-purity subgroups by measuring the relative contribution of the two types of transition base substitution (A>G/G>A and T>C/C>T) and the four classes of transversion base substitutions (C>A/A>C, C>G/G>C, T>A/A>T and T>G/G>T). Two of the ten TCGA data sets (head and neck squamous cell carcinoma, lung squamous cell carcinoma) showed a significantly decreased fraction of T>A substitutions in the low-purity group compared with the high-purity group (unpaired t- test with Benjamini–Hochberg FDR correction, adjusted P =0.015 and 0.015, respectively) ( Supplementary Table S5 ). The ratio of transitions and transversions was significantly associated with purity level in head and neck squamous cell carcinoma (adjusted P =0.018). We have developed a new algorithm to infer the level of infiltrating stromal and immune cells in tumour tissues and tumour purity using gene expression data. The predictive ability of this method has been validated in large and independent data sets. Genomic, transcriptomic and proteomic analyses using clinical tumour tissue are affected by the fraction of tumour cells present, and methods for evaluation of the non-tumour portions of tumour samples could provide an important context to genomic data analysis [15] . ESTIMATE scores were significantly correlated with the tumour purity of clinical cancer samples as well as cancer cell line samples and provide an accessible and straightforward approach to obtain a measure of the amount of tumour cells in a biological sample. The ESTIMATE algorithm may be further optimized by including signature of endothelial cells and tumour-type-specific normal epithelial cells. Tumour purity of clinical tumour samples is routinely determined by pathologists through visual evaluation of hematoxylin- and eosin-stained slides. In this study, histological estimates of the percentage of tumour cells, stromal cells and infiltrating lymphocytes did not correlate well with ESTIMATE, stromal and immune scores, consistent with the weak correlation between DNA copy number-based tumour purity and histological tumour purity [15] . This discrepancy between genomic- or transcriptomic-based and pathology-based estimates might be affected by the sensitivity of histopathological examination to interobserver bias and variability in accuracy [15] , [41] or the difference in tissue sections [42] in the same sample between nucleic acid extraction and histological evaluation. The contribution of immune cells to ovarian carcinoma is well recognized [5] , [6] , and we chose to use the TCGA ovarian carcinoma samples as the basis for development of the immune signature, as four types of principal information were available: tumour tissue for cell-sorting experiments, estimates of the amount of desmoplasia, immunohistochemistry-based counts of the number of leukocytes and methylation leukocyte scores. Importantly, the performance of ESTIMATE in both TCGA and non-TCGA ovarian carcinoma data sets was not distinctively better compared with other tumour types, and we thus believe that the method used to develop the signature is not biased towards ovarian cancers. The fibroblast/mesenchymal nature of stromal cells separates their gene expression profile from that of the epithelial tumour cells, thus providing a rationale to seek a signature that is characteristic of stromal cells in general, despite the notion that stromal cells may be tumour-type-specific. As expression data sets from three cancer types (ovary, breast and colon) were used to compare tumour cell fractions and matched stromal cell fractions after laser-capture microdissection, we suggest that some of the diversity in tumour-associated stroma among various cancer types was captured. Importantly, the ESTIMATE accuracy among ovarian, breast and colon cancer TCGA samples was not notably better than that of other tumour types, suggesting that the stromal signature can be broadly applied. The dependency of ESTIMATE on infiltrating stromal and immune cells resulted in some limitations, such as the inability to accurately infer tumour cellularity of hematopoietic or stromal tumours (for example, leukaemia, sarcoma and gastrointestinal stromal tumours) because of the high and tumour-intrinsic expression of stromal- or immune-related genes. Owing to the lack of data, we were unable to evaluate ESTIMATE in the context of tumour types such as prostate or pancreas cancer that may present with atypical patterns of tumour-associated cells—that is, increased fractions of normal epithelial cells. Additional methods may be needed to predict cancer cell fractions for such malignancies. The diverse pattern of the presence of stroma and immune cells across tumour types further emphasizes the different context-dependent ways in which tumour-associated normal cells function and more broadly illustrates the impact of the tumour microenvironment on tumorigenesis and homeostasis. Epithelial-to-mesenchymal transitions in tumour cells have been frequently described [43] . It is possibility that some overlap exists between the stromal expression signature and a mesenchymal tumour cell phenotype. However, the strong correlation with tumour purity may suggest that epithelial-to-mesenchymal transition is often confused with the increased presence of tumour-associated stroma. Low tumour purities may reduce the sensitivity of somatic mutation detection [44] . We did not observe an association of tumour purity with mutation rates except in head and neck squamous cell carcinomas and clear cell renal cell carcinoma, suggesting that the impact of tumour purity to identify somatic mutations is less compared with other factors such as depth or coverage or the mutation detection algorithm applied. We noted differences in mutational profile and spectrum between high and low stromal/immune subgroups in several tumour types. The consistent reduction in T>A substitutions in some low-purity cases suggests that the tumour microenvironment can have an impact on mutational processes or alternatively that the types of mutations in the tumour can alter stromal and immune infiltrations. Our ESTIMATE method for the assessment of stromal and immune cells in tumour tissues may provide an additional avenue to increase our understanding of molecular phenotype. Our results show that the levels of stromal and immune cells in tumour tissue can be associated with clinical characteristics. Further refinement of the lineage characteristics of infiltrating cells, such as distinguishing between various types of leukocytes, may reveal a more consistent pattern of clinical associations than what we have currently described. Novel therapeutics such as ipilumimab and nivolumab alters T-lymphocyte checkpoint control and may be particularly effective in tumours with intrinsically high levels of infiltrating leukocytes. Whether ESTIMATE immune scores could serve as a biomarker for immunotherapy response is a topic for further investigation. The ESTIMATE method can be applied for assessment of the presence of stromal cells and the infiltration of immune cells in tumour samples using gene expression data. The method is publicly available through the SourceForge software repository ( https://sourceforge.net/projects/estimateproject/ ). The application of ESTIMATE to publicly available microarray expression data sets, as well as new microarray or RNA-seq-based transcriptome profiles, may help in elucidating the facilitating roles of the microenvironment to neoplastic cell and provide new insights into context in which genomic alterations occur. Data preparation TCGA level 3 gene expression levels were obtained from the TCGA Data Portal [45] in March 2013. In this study, we used 10 tumour types from four platforms: Affymetrix HT-HG-U133A (one-colour type—that is, one RNA sample is labelled with a fluorophore and hybridized to a microarray), Agilent G4502A (two-colour type—that is, one sample and one reference are labelled with different fluorophores and hybridized together on a same microarray), RNAseq (quantified as Reads Per Kilobase per Million mapped reads) [46] and RNAseqV2 (quantified through RNA-seq by Expectation Maximization) [47] ( Table 1 ). The tumour types selected for our study were among the first tumour types analysed through TCGA and were selected as cancer types studied in TCGA’s Pan-Cancer project. In addition, we used 31 data sets of microarray expression or SNP array copy numbers from Gene Expression Omnibus [48] and ArrayExpress [49] , glioblastoma expression data set from the Repository of Molecular Brain Neoplasia Data [50] , cancer cell line expression data set from Cancer Cell Line Encyclopedia (CCLE) [51] and a glioma stem-like cell expression data set from researchers at MD Anderson Cancer Center ( Supplementary Table S1 ). Microbead-based cell sorting First, the tissue of a fresh frozen ovarian cancer sample was diced into 1-mm pieces. The tissue was further enzymatically dissociated with 0.8 mg/ml HBSS Liberase Research Grade (#05-401-119-001; Roche) and incubated at 37 °C for 1 h, followed by mechanical dissociation using an 18-G needle. To isolate single cells, the resulting cell suspension was filtered using a 40-μm filter. Lastly, the remaining cells were separated into an epithelial tumour cell fraction and a non-epithelial tumour-associated stromal fraction. For cell sorting, we used antibody-coated microbeads that recognize the epithelial cell surface marker EpCAM (#130-061-101; Miltenyi Biotec), which results in an EpCAM-positive tumour cell fraction and an EpCAM-negative tumour-associated stromal cell fraction. To test the efficiency of our procedure we performed gene expression profiling on three bulk tumours, three EpCAM-positive fractions and three EpCAM-negative fractions after cell sorting using Illumina BeadChip Human HT-12 v4 according to the manufacturer’s instructions. This study was approved by the institutional ethics review board at The University of Texas MD Anderson Cancer Centre (Lab 07-0108). All patients provided written informed consent for the collection of samples and subsequent analysis. Microarray data processing Probes from Affymetrix HG-U133A, HG-U133Plus2.0 and HT_HG-U133A GeneChip platforms were mapped to a transcript database and combined in one probe set per gene, as described previously [52] . Expression levels from these Affymetrix data sets were individually established using RMA and quantile normalization [53] . Raw data from Affymetrix Human 133 × 3 P array were processed using the Bioconductor rma package with the default setting. On the Agilent G4112F platform, data normalization was carried out in GeneSpring GX 11.5 (Agilent Technologies) by setting the raw signal threshold to 1.0 and using 75th percentile normalization [54] . Quantile normalization was performed for Illumina Human HT-12 v4 microarray data using the Bioconductor preprocessCore package. On Affymetrix Human 133 × 3P array, Agilent G4112F and Illumina Human HT-12 v4 probes measuring the same gene were averaged to obtain one expression value per gene and sample. Gene selection A flowchart of gene selection in this study is shown in Supplementary Fig. S1 . To analyse expression data measured from six different platforms, we extracted 10,412 common genes. In the gene selection process, we used the significance analysis of microarray [55] method to detect differentially expressed genes (more than twofold and q <0.0001) between two groups. First, by comparing normal hematopoietic cells (two CD14 monocytes, two dendritic cells, two CD56 NK cells, two CD4 T-cells, two CD8 T-cells and two CD19 B-cells) to other normal cells in the GSE1133 data set, we divided 10,412 common genes into two groups: 1,222 genes that were upregulated in normal hematopoietic cells (named ‘normal hematopoietic cell-related genes’) and 9,190 other genes. Second, to extract genes associated with infiltrating immune cells in tumour tissues, we adopted leukocyte methylation signature scores that describe the level of immune cell infiltration in ovarian cancer tissues using methylation data [15] . Of 489 samples in TCGA ovarian cancer-unified expression data [56] , 403 samples include a leukocyte methylation signature score. We defined the respective high and low immune cell infiltration groups as those having a leukocyte score higher than the 97th percentile ( n =14) and those with a score lower than the 3rd percentile ( n =14). We compared the two groups. As a result, we extracted 447 upregulated genes in the high immune cell infiltration group and found 161 genes that overlapped between the 1,222 normal hematopoietic cell-related genes and the 447 genes related to infiltrating immune cell-related genes. Third, we compared the tumour portion with their matched stromal part after laser-capture microdissection including ovarian cancer (GSE9890), breast cancer (GSE14548) and colorectal cancer (GSE35602) in order to evaluate the possibility that stroma-forming cells in tumour tissue differ among various tumour types. For those three respective data sets, we extracted 245, 300 and 1,147 upregulated genes in stromal samples and picked up 338 stromal-related genes that overlapped in at least two data sets. Fourth, to exclude genes with high variability across tumour types, we calculated the median absolute deviation (MAD) based on 451 samples from the CCLE expression data set, which consisted of breast, brain, colon, endometrial, kidney, lung and ovarian cancer types. We defined genes with MAD <0.5 as genes with low variability [13] in the CCLE data set and selected 172 overlapping genes related to the presence of stroma in tumour tissue samples. Furthermore, as brain tumours are derived from non-epithelial cells, brain tumours highly express some stromal markers that have been previously reported. Therefore, we calculated the average expression level per gene and ranked the genes in the order of the average expression level in the glioma stem-like cell data set to exclude genes highly expressed in stromal tissue in brain tumours. We decided that genes ranked lower than the median rank as low expression in glioma stem-like cells. After that, we extracted 141 stromal genes. To unify the number of genes between those related to stroma and to immune cell infiltration, we extracted 141 genes related to immune cell infiltration by selecting the top-ranked 141 genes after sorting by the significance analysis of microarray score obtained by comparison of the high to low immune cell infiltration groups. Genes included in the two signatures are listed in Supplementary Data 1 . In the evaluation of the two signatures across the TCGA data sets, we observed that the stromal signature prior to including the two additional filtering steps was not able to provide equivalent predictive ability compared with that of the immune signature. As tuning the signature based on its performance in the TCGA data sets of other tumour types increased the risk of overfitting, we validated the effectiveness of the signatures on the independent data set ( Fig. 4b ; Supplementary Fig. S8c ). ESTIMATE ESTIMATE outputs stromal, immune and ESTIMATE scores by performing ssGSEA [13] , [23] , [37] . For a given sample, gene expression values were rank-normalized and rank-ordered. The empirical cumulative distribution functions of the genes in the signature and the remaining genes were calculated. A statistic was calculated by an integration of the difference between the empirical cumulative distribution function, which is similar to the one used in gene set-enrichment analysis but based on absolute expression rather than differential expression. We defined ssGSEA based on the signatures related to stromal tissue and immune cell infiltration as stromal and immune scores and combined the stromal and immune scores as the ‘ESTIMATE score’. The formula for calculating ESTIMATE-based tumour purity was developed in TCGA Affymetrix data ( n =1,001) including both the ESTIMATE score and ABSOLUTE-based tumour purity. To develop a precise prediction model for tumour purity, we excluded six outliers from all Affymetrix data by computing a multivariate outlier criterion based on the generalized extreme studentized deviate test [57] , [58] using the Bioconductor Parametric and Resistant Outlier Detection (PARODY) package ( Supplementary Fig. S8a ). Next, we entered both the ESTIMATE score and tumour purity to Eureqa Formuliza 0.97 Beta using the default setting [59] . Eureqa attempts to design a mathematical formula that fits observed data employing an evolutionary algorithm [60] . We obtained a fitted formula to predict tumour purity based on the ESTIMATE score. Finally, we applied this formula to the nonlinear least squares method (nls function for stats package) to determine the final formula for predicting tumour purity, as follows: Tumour purity=cos (0.6049872018+0.0001467884 × ESTIMATE score). (1) HAPSEG and ABSOLUTE ABSOLUTE-based tumour purity in the TCGA data sets was obtained from each TCGA working group. To calculate ABSOLUTE-based tumour purity in other data sets, we ran HAPSEG version 1.1.1 and ABSOLUTE version 1.0.4. As indicated on the website [61] , we ran Birdseed v1 using Affymetrix Power Tools [62] and input the resulting apt-probeset-summarize and apt-probeset-genotype files into HAPSEG. After that, we ran ABSOLUTE at the default setting. In the subsequent analyses, we used samples for which the tumour purity levels were called by ABSOLUTE. SNP array data for HAPSEG and ABSOLUTE We downloaded SNP array data from Gene Expression Omnibus [48] and ArrayExpress [49] . We used Affymetrix CEL files (including per-probe intensity values) from two platforms (Affymetrix GeneChip Human Mapping 250 K Sty array and Genome-Wide Human SNP array 6.0) in this study. Samples that had passed the 93% call-rate threshold (GeneChip Human Mapping 500 K array) or the 86% threshold (Genome-Wide Human SNP array 6.0) [63] were applied to the ABSOLUTE algorithm [15] . Leukocyte methylation score We downloaded leukocyte methylation score data (syn1809223) [15] that predicts the fraction of leukocyte in tumour tissue based on genome-wide DNA methylation data from Synapse BETA [64] and investigated the correlation of stromal, immune and ESTIMATE scores with leukocyte methylation scores for each tumour type. Histological purity estimates We downloaded Biotab clinical information per sample from the TCGA Data portal. Basically, each tumour specimen was embedded in optimal cutting temperature medium, and histologic sections were obtained as top and bottom portions for pathological review. Of ‘biospecimen_slide’ data for each tumour type, we used ‘percentage of infiltrating lymphocyte’, ‘percentage of stromal cells’ and ‘percentage of tumour cells’ to examine the association of our stromal, immune and ESTIMATE scores and histological findings. For samples with multiple slide data, we used the mean of each value in performing correlation analysis. Mutation analysis We downloaded mutation annotation format files (syn1710680) and mutation rates (syn1713813) based on MuSIC [65] for 10 different types of tumours from Synapse BETA [64] . From the mutation annotation format files, we extracted mutation status for 10,412 common genes that were used as background in the ESTIMATE algorithm. Of the several mutation types, we used ‘Frame_Shift_Del/Ins,’ ‘In_Frame_Del/Ins,’ ‘Missense_Mutation’ and ‘ Nonsense_Mutation’ in this study. We converted the mutation status per gene that was converted into binary data (1, mutated; 0, wild type) to use in the mutation analysis. To examine the impact of infiltrating normal cells on genetic alterations, we extracted high and low ESTIMATE score subgroups from the expression data per tumour type. The high and low ESTIMATE score subgroups were defined, respectively, as samples with scores higher than the 75th percentile and within the 25th percentile of the ESTIMATE score range. We combined the expression data in the two subgroups with somatic mutation binary data. Samples without either expression or mutation were excluded from this analysis. Mutation frequency was evaluated by the number of mutations per Mbp [26] , [27] , [28] , [29] . To investigate the mutation spectrum between the two subgroups per tumour type, we selected single-nucleotide alterations and converted them into the six classes of base substitution (C>A, C>G, C>T, T>A, T>C and T>G) [66] , [67] . We then calculated the relative contribution of each of the six classes of base substitutions and compared them between the two subgroups. Next, we extracted the respective high and low stromal/immune score subgroups based on the 75th and 25th percentiles of each score per tumour type and combined each subgroup’s expression data and mutation data. Statistical analysis We conduced all computations with R 2.13.2 (ref. 68 ) and used standard statistical tests as appropriate. Where appropriate, P -values were corrected for multiple testing using the Benjamini–Hochberg false discovery rate method [69] . How to cite this article: Yoshihara, K. et al. Inferring tumour purity and stromal and immune cell admixture from expression data. Nat. Commun. 4:2612 doi: 10.1038/ncomms3612 (2013).